Coordination-driven self-assembly of a molecular figure-eight knot and other topologically complex architectures Over the past decades, molecular knots and links have captivated the chemical community due to their promising mimicry properties in molecular machines and biomolecules and are being realized with increasing frequency with small molecules. Herein, we describe how to utilize stacking interactions and hydrogen-bonding patterns to form trefoil knots, figure-eight knots and [2]catenanes. A transformation can occur between the unique trefoil knot and its isomeric boat-shaped tetranuclear macrocycle by the complementary concentration effect. Remarkably, the realization and authentication of the molecular figure-eight knot with four crossings fills the blank about 4 1 knot in knot tables. The [2]catenane topology is obtained because the selective naphthalenediimide (NDI)-based ligand, which can engender favorable aromatic donor-acceptor π interactions due to its planar, electron-deficient aromatic surface. The stacking interactions and hydrogen-bond interactions play important roles in these self-assembly processes. The advantages provide an avenue for the generation of structurally and topologically complex supramolecular architectures. Scientists’ interest in complicated molecular knots, links, and entanglements has grown rapidly in recent decades [1] , [2] , [3] , [4] , [5] . Naturally occurring DNA knots were first discovered in 1967 [6] , [7] , and nearly a decade later, circular DNA-containing links were reported [8] . Carbonic anhydrase was the first identified protein with a knotted tertiary structure, a finding published in 1977 [9] . Recently, AFM imaging was employed to unequivocally illustrate the catenane and trefoil knot structures of polymer molecules [10] . While knots and links have particular relevance in the field of biology, they also have been the subject of significant advances in chemical topology. The first nontrivial molecular knot, a trefoil knot [11] , was synthesized by Sauvage using a metal template strategy, along with a Solomon link [12] . Examples of figure-eight knots [13] , pentafoil knots [14] , [15] , [16] , [17] , 8 19 knots [18] , and 8 18 knots [19] have since been successfully synthesized. Recently, the realization of a + 3 1 # + 3 1 # + 3 1 composite knot [20] and a granny knot [21] have pushed new boundaries in the synthesis of complicated knots. Although a number of trefoil knots (3 1 ) [22] , [23] , [24] , [25] , [26] , [27] , [28] have been prepared to date, there are few works providing an insight into the transformation between monomeric macrocycles, molecular knots and links. In addition, in contrast with trefoil knots, figure-eight knots (4 1 ) are exceedingly rare. Only one likely synthesis of a molecular figure-eight knot (4 1 ) exists, provided by the group of Sanders, the structure of which was determined based largely on symmetry and NMR data [13] . And that the representation of 4 1 knot is eight crossings rather than four crossings by additional four nugatory crossings [3] . To date no single-crystal structure exists of either a synthetic molecular figure-eight knot or the reduced representation with four crossings, thus our understanding of molecular figure-eight knots remains rudimentary. Thus, constructing and authenticating such a species remains a formidable challenge in the field of supramolecular chemistry. In recent years, the organometallic half-sandwich fragments [Cp*M] (M = Ir, Rh; Cp* = η 5 -pentamethyl-cyclopentadienyl) and [Ru( p -cymene)] have emerged as versatile building blocks for the construction of supramolecular compounds such as molecular Borromean rings [29] , molecular Solomon links [30] , Hopf’s links [31] , and so on. Herein, we report the coordination-driven self-assembly [31] , [32] , [33] , [34] , [35] , [36] , [37] of monomeric macrocycles, trefoil knots, figure-eight knots, and [2]catenanes by the combination of flexible ester ( L1 ) and amide ( L2 ) ligands with [Cp*M] (M = Ir, Rh) organometallic connecting units. Interestingly, the transformation between monomeric macrocycles, trefoil knots and links is effected by merely changing the size of the side arms units. The realization and authentication of a molecular figure-eight knot presented herein is an inspiring and long-awaited achievement. A careful study of single-crystal structure of the knot indicates that the molecule can adopt various forms by altering its conformation, including the reduced form with four crossings and the four-fold symmetry form with eight crossings (Fig. 1 ). These synthesized knots and links are unambiguously characterized by NMR spectroscopy, ESI-MS, and single-crystal X-ray diffraction analysis. Furthermore, density functional theory (DFT) calculations are used to provide insight into the formation of the [2]catenane and trefoil knots. Fig. 1 The macrocycles, molecular knots and links prepared in this study with their trivial names and descriptors using the Alexander–Briggs notation [38] . a 0 1 Unknot, ( b ) 3 1 Trefoil knot ( c ) 4 1 Figure-eight knot and ( d ) [2]Catenane Full size image Selection of ligands The flexible ligands 1,4-phenylenebis(methylene) diisonicotinate ( L1 ) and N,N′-[1,4-phenylenebis-(methylene)]bis-4-pyridinecarboxamide ( L2 ) were chosen because of the high degrees of rotational freedom of its ester and amide functional groups, which can allow the ligand to present a variety of configurations and induce hydrogen-bond interactions. In addition, its π-conjugated phenyl and pyridyl moieties can engender favorable aromatic π–π stacking and CH–π interactions [39] , [40] , [41] . The stacking interactions and hydrogen bonding interactions can be considered as the driving force for the formation of trefoil knot and figure-eight knot, while a [2] catenane was formed by the combination of another planar, electron-deficient aromatic edge unit ( E4 ) with L1 . Self-assembly of a tetranuclear macrocycle and trefoil knot The reaction of [Cp*RhCl 2 ] 2 with AgOTf (2.0 equiv), followed by the addition of L1 , produced chair-shaped tetranuclear macrocycle complex 1 (yield: 92%) (Supplementary Fig. 12). The structure of 1 was confirmed by electrospray ionization mass spectrometry (ESI-MS), 1 H NMR spectroscopy, and X-ray crystallographic analysis (Supplementary Fig. 1). The ESI-MS data of 1 in CH 3 OH shows a peak at 2235.04 m / z assigned to [ 1 –OTf – ] + , indicating that complex 1 is stable in solution (Supplementary Fig. 50). Upon treating flexible ligand L1 with the longer edge unit E2 in a 1:1 molar ratio, a yellow mixture was obtained in a total yield of 90% (Fig. 2 ), which was studied by NMR spectroscopy in CD 3 OD (Fig. 3 ). Fig. 2 Synthesis of tetranuclear macrocycle 2a and trefoil knot 2b . Schematic representation of the synthesis of E2 and the stick model of E2 ; Schematic representation and stick model of L1 ; Increasing the concentration of 2a can result in gradual transformation of 2a into 2b Full size image Fig. 3 1 H NMR spectrum (400 MHz, CD 3 OD) of 2b ( a ), 2a + 2b ( b ), and 2a ( c ). DOSY spectrum (500 MHz, CD 3 OD) of 2a + 2b ( d ), (The peaks at 3.50 and 1.18 ppm belong to diethyl ether) Full size image Diffusion-ordered NMR spectroscopy (DOSY) indicated the presence of two diffusion coefficients ( D = 4.7 × 10 −10 m 2 s −1 ( 2a ) and 2.8 × 10 −10 m 2 s −1 ( 2b )), suggesting the existence of two different compounds in the reaction mixture (Fig. 3 ). Increasing the concentration of 2a + 2b in CD 3 OD from 2.0 mM to 32.0 mM (with respect to Cp*Rh; Supplementary Fig. 28) led to gradual transformation of the tetranuclear complex 2a into trefoil knot 2b . At a low concentration (2.0 mM), only 2a was observed in solution (Supplementary Fig. 18). When in a saturated solution (32.0 mM), 2a was almost entirely converted to 2b (90.6 mass%) based on 1 H NMR spectroscopy (Supplementary Fig. 21). The 1 H NMR signals of the phenyl and benzyl protons of 2b showed large upfield shifts to 2.0–4.5 ppm, indicating the tight π–π stacking of phenyl groups. To further study the contribution of π–π stacking interactions to the formation of 2b , the π-electron-rich guest molecule pyrene was added into the mixture of 2a + 2b . Upon addition of increasing amounts of pyrene (from 0 to 6 equiv), the mixture was converted to the pure monomeric macrocycle 2a based on 1 H NMR spectroscopy (Supplementary Fig. 32). Based on the established hydrophobic properties of these macrocycles [42] , [43] , [44] , D 2 O was added gradually to the 12.0 mM CD 3 OD solution of 2a + 2b . The resulting 1 H NMR spectrum showed that upon changing the solvent ratio (CD 3 OD:D 2 O, v/v) from 7:0 to 7:7, the mixture of 2a + 2b underwent nearly complete transformation to the trefoil knot 2b (Supplementary Fig. 33). In addition, a 1 H NMR spectrum in DMSO showed that the vast majority of the complex existed in the monomeric macrocycle 2a form over a wide concentration range (8.0–24.0 mM, with respect to Cp*Rh; Supplementary Fig. 34). Along with this NMR spectroscopic data, ESI-MS also indicated the presence of two complexes in solution: [ 2a –OTf – ] + ( m/z = 2559.27) (Supplementary Fig. 51) and [ 2b –2OTf – ] 2+ ( m/z = 1882.24) (Supplementary Fig. 52). Single crystals suitable for X-ray diffraction were obtained by slow vapor diffusion of diethyl ether into a methanol solution of 2a and 2b , in order to unambiguously confirm the structure and topology of 2a and 2b . The solid-state structure of complex 2a was confirmed by single-crystal X-ray diffraction analysis to be a boat-shaped tetranuclear macrocycle. Interestingly, the structure is unsymmetrical, with dimensions of 5.60 Å (short Rh ∙∙∙ Rh nonbonding distance; Fig. 4 ), 13.69 and 15.01 Å (long Rh ∙∙∙ Rh nonbonding distances; Fig. 4 ). The distance between the two phenyl groups of L1 is 7.13 Å, which is even longer than the short Rh ∙∙∙ Rh nonbonding distance of E2 , indicating that there is no π–π stacking interactions between the phenyl groups. Fig. 4 Single-crystal X-ray structure of 2a . Top view ( a ), side view ( b ), and front view ( c ). Counteranions and hydrogen atoms are omitted for clarity (N, blue; O, red; C, gray; Rh, purple) Full size image The crystal structure of 2b was refined in the C12/c1 space group, revealing the complex to have the topology 3 1 according to the Alexander–Briggs notation [38] . The right-handed trefoil knot + 3 1 has three positive crossings [3] , [11] , [24] , and a highly symmetrical main framework of point group C 3 . The mirror-image symmetric isomeric topology –3 1 exists in the same cell in a 1:1 molar ratio. Left-handed trefoil knot –3 1 has three negative crossings, and a highly symmetrical main framework with the same point group C 3 (Supplementary Fig. 4). The ligand arms E2 and L1 , which are connected by Rh atoms, form a main framework consisting of two triangles, with dimensions of 14.76 and 5.57 Å (Rh ∙∙∙ Rh nonbonding distances; Fig. 5 ). The average outer diameter of the structure is 24.4 Å and the average inner diameter is 4.8 Å (a circle bound by the inner three O atoms; Fig. 5 ). A close-contact analysis of the structure shows that the trefoil knot is stabilized by parallel-displaced π–π interactions (of interlayer distance 3.38 Å) between the pyridyl moieties and phenyl moieties of three ligands L1 , as well as edge-to-face-type CH–π interactions (2.66 Å) between BiBzIm moieties and phenyl moieties (Supplementary Fig. 2). Moreover, in the solid state, intermolecular hydrogen bonds exist between the O atoms of the ester units and the Cp* protons of another contiguous molecular knot, in the range of 2.51 to 2.67 Å (Supplementary Fig. 3). 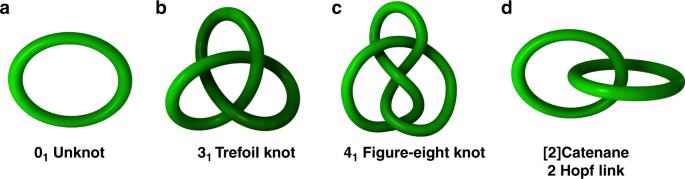Fig. 1 The macrocycles, molecular knots and links prepared in this study with their trivial names and descriptors using the Alexander–Briggs notation38.a01Unknot, (b) 31Trefoil knot (c) 41Figure-eight knot and (d) [2]Catenane In order to gain insight into the formation of 2b , DFT binding energy calculations were performed to study the intermolecular interactions in 2b (trefoil knot; Supplementary Table 1). The energy of formation of the trefoil knot structure from three monomers of 2_3mo (monomer like 4 ; Supplementary Fig. 56) was calculated to be −76.0 kcal/mol, while the contribution energy of π–π stacking was found to be −53.9 kcal/mol. Fig. 5 Single-crystal X-ray structure of 2b . Top view ( a ) and side view ( b ). Counteranions and hydrogen atoms are omitted for clarity Full size image Self-assembly of a figure-eight knot (3) The generation of the trefoil knot 2b gave us great inspiration, in that stacking interactions and intermolecular hydrogen bonds interactions clearly play synergistic roles in the formation of organometallic knots. Given this realization, in the place of ester-containing ligand L1 , we decided to employ the amide-containing ligand L2 . We speculated that the amide groups of L2 would provide additional means of hydrogen bonding due to the presence of the N–H group, enabling the construction of amide-amide H-bonds and perhaps leading to more extensive hydrogen bonding and more complicated structures. A yellow solid 3 (yield: 82%) was obtained by treating amide ligand L2 with edge unit E2 in a 1:1 molar ratio (Fig. 6 ), and the structure of 3 was confirmed by NMR spectroscopy, ESI-MS, and single-crystal X-ray diffraction analysis. Fig. 6 Synthesis of octanuclear figure-eight knot 3 . Schematic representation of the synthesis of 3; The stick model (top) and schematic representation (below) of E2 and L2 ; The stick model (top) and simplified image of 3 Full size image The 1 H NMR spectrum of 3 in CD 3 OD exhibits two sharp Cp* singlets at δ = 1.771 and 1.683 ppm in a ratio of 1:1, corresponding to two disparate Cp*Rh environments, which may signify the existence of a specific topological structure. Furthermore, some signals in the 1 H NMR spectrum of 3 are shielded with respect to those of building block E2 , reflecting the compact structure of the molecule, in which each region of the loop is in close proximity with aromatic rings (Supplementary Fig. 35). The 1 H DOSY NMR spectrum of 3 (Supplementary Fig. 38) showed that the aromatic and Cp* signals were associated with a single diffusion constant, suggesting that only one stoichiometry of assembly was formed. The structure of 3 in solution was also supported by ESI-MS. The prominent peaks at m / z = 2555.44 ([3−2OTf – ] 2+ ) is in good agreement with their theoretical distribution (Supplementary Fig. 53), suggesting that the structure remains intact in solution. The 1 H NMR signals did not change over a wide concentration variation range (2.0–12.0 mM, with respect to Cp*Rh, Supplementary Fig. 39), indicating a compact and stable structure. Single crystals of 3 were obtained by slow diffusion of diethyl ether vapor into a solution of 3 in methanol and the solid-state structure was determined by X-ray diffraction analysis. The crystal structure of 3 was refined in the I4 1 /a space group. The crystal structure unequivocally confirmed the topology of the molecular 4 1 knot according to the Alexander–Briggs notation [38] . (Fig. 7 ) show the reduced form of the 4 1 knot comprising four crossings. When viewing the structure 3 in the c direction, the molecular knot 3 is highly symmetrical and has a rotary inversion axis ( S 4 ), which means that a rotation of 90° converts this representation into its mirror image, thereby making it achiral (Fig. 7 ). Fig. 7 Single-crystal X-ray structure of 3 . The reduced representation with four crossings ( a ) and the four-fold symmetry representation ( c ) of 3 , and simplified structures of the reduced representation with four crossings ( b ) and the four-fold symmetry representation ( d ) of 3 in which sticks connect the rhodium centers Full size image As in trefoil knot structure 2b , E2 , and L2 , which are connected by Rh atoms, form a closed loop with four nonalternating crossings. Close-contact analysis of the structure reveals a figure-eight knot arrangement similar to a tetrahedral configuration, held together by both edge-to-face-type CH–π interactions (3.39 Å) and parallel-displaced π–π interactions (of interlayer distance 3.72 Å) between phenyl moieties and relatively adjacent two pyridyl moieties of three L2 ligands. Unlike trefoil knot 2b , in which C–O … H intermolecular hydrogen bond interactions are formed between carbonyl oxygen atoms of the ester moieties and Cp* protons, the figure-eight knot 3 presents intramolecular N–H … O hydrogen bonding interactions (2.79 Å) between NH hydrogen atoms and carbonyl oxygen atoms from the amide moieties of two L2 ligands. These four intramolecular N–H … O hydrogen bonding interactions play a crucial role in the stabilization of a figure-eight knot (Supplementary Fig. 5). In addition, the analogous Cp*Ir-based 4 1 knot complex 3′ was separately constructed in a yield of 84% (Supplementary Fig. 6). In a word, the non-covalent interactions (NCIs), i.e., π–π stacking interactions, CH–π interactions and hydrogen bonding interactions, play synergetic roles in the formation of a figure-eight knot with four crossings. Self-assembly of binuclear trapezoidal macrocycle 4 In order to weaken the π–π stacking interactions between the pyridyl moieties and phenyl moieties in the trefoil knot structure, the longer ligand 2,5-dichloro-3,6-dihydroxy-1,4-benzoquinone (H 2 CA, L3 ) was deliberately chosen to build the edge unit E3 [Cp* 2 Rh 2 ( μ -CA)Cl 2 ] upon formation of the macrocycle. By direct reactions of E3 with ligand L1 , the binuclear trapezoidal macrocycle 4 was obtained in a 95% yield rather than a tetranuclear ring as in complex 1 (Supplementary Fig. 13), and the structure of 4 was confirmed by NMR spectroscopy, ESI-MS and single-crystal X-ray diffraction analysis (Supplementary Fig. 7). Self-assembly of [2]catenane 5 The parallel upper and bottom surfaces of 4 , as well as its cavity, prompted us to explore the synthesis of a molecular [2]catenane by employing an edge unit with a suitable electron-poor aromatic group. We speculated that favorable Donor-Acceptor stacking interactions between dinuclear edge unit E4 and the flexible ligand L1 may enable the self-assembly of a [2]catenane (Fig. 8 ). The length of the naphthalenediimide (NDI) edge unit is 11.9 Å [45] (Rh–Rh nonbonding distance), which is large enough to allow the phenyl group of the flexible ligand L1 to pass through. Fig. 8 Synthesis of [2]catenane complex 5 . Schematic representation of the synthesis of E4 (top) and stick model of 5 (below) Full size image As expected, the resulting [2]catenane complex 5 was formed in a yield of 93%, as revealed by NMR studies. The 1 H NMR spectrum of 5 showed that the benzyl proton resonance was split into two broad signals (Supplementary Fig. 44) rather than the single resonance previously observed in macrocycle 4 (Supplementary Fig. 40), indicating the existence of a stable topological structure. Partial variable-temperature 1 H NMR spectra of 5 showed that from 298 to 333 K, the split, broad signals of the NDI and benzyl groups merge into a single signal, suggesting that the [2]catenane topology limits the rotation of benzyl moieties on the 1 H NMR timescale (Supplementary Fig. 49). The 1 H DOSY NMR spectrum of 5 (Supplementary Fig. 46) showed that the aromatic and Cp* signals were associated with a single diffusion constant, suggesting that only one stoichiometry of assembly was formed. The ESI-MS data also indicated that complex 5 preserved its [2]catenane structure in solution: [ 5 –OTf – ] + ( m/z = 2687.20) (Supplementary Fig. 55). The proton signals remained unchanged over a wide concentration range (2.0–12.0 mM with respect to Cp*Rh; Supplementary Fig. 48), indicating that the Donor–Acceptor stacking interactions are strong enough to maintain the [2]catenane topology even in dilute solutions. This phenomenon contrasts with those observed in recent studies on [2]catenane structures [31] , [46] , [47] . The X-ray structure of 5 confirmed its [2]catenane structure (Fig. 9 ), wherein two catenated trapezoids make up an inseparable ensemble. As expected, [2]catenane 5 is stabilized by strong π–π stacking interactions (3.44 Å, Fig. 9 ) between the NDI moieties of E4 and the phenyl moieties of L1 . In addition, there are no π–π stacking interactions between the phenyl moieties, the inter-ring distances being 4.84 Å (Fig. 9 ), much larger than the normal π–π stacking distance (~3.5 Å). 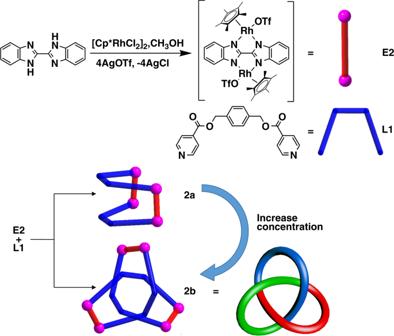Fig. 2 Synthesis of tetranuclear macrocycle2aand trefoil knot2b. Schematic representation of the synthesis ofE2and the stick model ofE2; Schematic representation and stick model ofL1; Increasing the concentration of2acan result in gradual transformation of2ainto2b In order to gain insight into the formation of 5 , DFT binding energy calculations were performed to study its intermolecular interactions (Supplementary Table 2). The energy of formation of the [2]catenane structure from two monomers of 4_3mo (monomer like 4 , Supplementary Fig. 59) was evaluated to be −30.5 kcal/mol, while the contribution energy of π–π stacking was found to be −41.4 kcal/mol. Fig. 9 X-ray structure of 5 ([2]catenane). a , b depictions of the short and long arms (N, blue; O, red; C, gray; Rh, purple) ( c ) ball-and-stick representations. Counteranions are omitted for clarity Full size image Transformations between monomeric macrocycles, molecular trefoil knots, and links are achieved by combining flexible ester ligand L1 with different carefully chosen edge units through coordination-driven self-assembly. Above all, by employing amide ligand L2 , a tetrahedral figure-eight knot comprising four crossings is realized, the solid-state structure of which shows that the molecule could display various forms, including a reduced representation with four crossings and a four-fold symmetry representation with eight crossings, merely by changing its conformation. In conclusion, the π–π stacking, CH–π interactions, and hydrogen bonding interactions play synergistic roles in the formation of molecular trefoil knot and figure-eight knot. Our results thus demonstrate a controllable all-in-one approach for the creation of molecular knots and links through supramolecular interactions [1] , [2] , [25] , [48] , which we hope will further inspire the strategic design of topologically complex molecular architectures, molecular machines, and functional nanodevices. Materials All reagents and solvents were purchased from commercial sources and used as supplied unless otherwise mentioned. The starting materials [Cp*RhCl 2 ] 2 and [Cp*IrCl 2 ] 2 (Cp * = η 5 -pentamethylcyclopentadienyl) [49] , BiBzIm (BiBzIm = 2,2´-bisbenzimidazole) [50] , and 2,7-dihydro-xybenzo[ lmn ][3,8]phenanthroline-1,3,6,8-( 2 H,7 H )-tetraone (DHNDI) [43] were prepared by literature methods. Characterization NMR spectra were recorded on Bruker AVANCE I 400 and VANCE-DMX 500 spectrometers. Spectra were recorded at room temperature. Chemical shifts are reported relative to the solvent residual peaks ( δ H = 3.31 (CD 3 OD)) or the solvent itself ( δ C = 49.00 (CD 3 OD)). Coupling constants are expressed in Hertz. Elemental analyses were performed on an Elementar Vario EL III analyzer. IR spectra of the solid samples (KBr tablets) in the range 400–4000 cm −1 were recorded on a Nicolet AVATAR-360IR spectrometer. ESI-MS spectra were recorded on a UHR TOF LC/MS mass spectrometer using electrospray ionization. Synthesis of 2a and 2b AgOTf (123.2 mg, 0.48 mmol) was added to a solution of [Cp*RhCl 2 ] 2 (74.0 mg, 0.12 mmol) in CH 3 OH (20 mL) at room temperature. The reaction mixture was stirred in the dark for 24 h and then filtered. BiBzIm (28.0 mg, 0.12 mmol) was added to the filtrate. The mixture was stirred at room temperature for 12 h to give a yellow solution. L1 (41.6 mg, 0.12 mmol) was then added. The mixture was stirred at room temperature for another 12 h to give a yellow solution. The solvent was concentrated to about 8 mL. Upon addition of diethyl ether, a yellow solid was precipitated and collected. The product was recrystallized from a CH 3 OH/diethyl ether mixture to afford a mixture of sheet-shaped crystals (2a) and needle-shaped crystals (2b). Characterization data for 2a and 2b : 146.4 mg, total yield of crystals: 90%. 2a (monomeric tetranuclear macrocycle) 1 H NMR (400 MHz, CD 3 OD, ppm, 2.0 mM, with respect to Cp*Rh): δ = 8.61 (d, J = 6.4 Hz, 8 H, pyridyl-αH), δ = 8.03 (q, J = 3.2 Hz, 8 H, BiBzIm-H), δ = 7.59 (d, J = 6.4 Hz, 8 H, pyridyl-βH), δ = 7.52 (q, J = 3.2 Hz, 8 H, BiBzIm-H), δ = 7.25 (s, 8 H, phenyl-H), δ = 5.30 (s, 4 H, benzyl-H), δ = 1.78 (s, 60 H, Cp*-H). Anal. Calcd for C 112 H 108 F 12 Rh 4 N 12 O 20 S 4 ( M = 2708.27): C, 49.64; H, 4.02; N, 6.20. Found: C, 49.45; H, 3.89, N, 6.12. 2b (trefoil knot) 1 H NMR (400 MHz, CD 3 OD, ppm, 32.0 mM, with respect to Cp*Rh, saturated): δ = 8.71 (d, J = 6.0 Hz, 12 H, pyridyl-αH), δ = 8.19 (d, J = 8.8 Hz, 6 H, BiBzIm-H), δ = 8.12 (d, J = 8.8 Hz, 6 H, BiBzIm-H), δ = 7.52 (m, 6 H, BiBzIm-H), δ = 7.29 (d, J = 6.4 Hz, 12 H, pyridyl-βH), δ = 4.49 (d, J = 13.2 Hz, 6 H, phenyl-H), δ = 4.21 (s, 12 H, benzyl-H), δ = 2.40 (d, J = 13.2 Hz, 6 H, phenyl-H), δ = 1.75 (s, 90 H, Cp*-H). 13 C{ 1 H} (101 MHz, CD 3 OD, ppm): δ = 8.45 (Cp*), δ = 97.56 (d, J = 7.7 Hz, Cp*), 64.07, 116.09, 116.44, 123.20, 123.63, 123.71, 125.62, 129.72, 133.36, 138.04, 143.42, 153.84, 155.85, 162.03. IR (KBr disk, cm −1 ): v = 1734, 1606, 1451, 1415, 1378, 1355, 1278, 1224, 1158, 1123, 1058, 1031, 966, 911, 856, 809, 774, 764, 755, 697, 638, 573, 518, 495, 440. Anal. Calcd for C 168 H 162 F 18 Rh 6 N 18 O 30 S 6 (M = 4062.41): C, 49.64; H, 4.02; N, 6.20. Found: C, 49.55; H, 3.86, N, 6.13. Synthesis of 3 (figure-eight knot) AgOTf (123.2 mg, 0.48 mmol) was added to a solution of [Cp*RhCl 2 ] 2 (72.0 mg, 0.12 mmol) in CH 3 OH (16 mL) at room temperature. The reaction mixture was stirred in the dark for 24 h and then filtered. BiBzIm (28.0 mg, 0.12 mmol) was added to the filtrate. The mixture was stirred at room temperature for 12 h to give a yellow solution. L2 (41.6 mg, 0.12 mmol) was then added. The mixture was stirred at room temperature for another 12 h to give a yellow solution. The solvent was concentrated to about 7 mL. Upon the addition of diethyl ether, a yellow solid was precipitated and collected. The product was recrystallized from a CH 3 OH/diethyl ether mixture to afford a block-shaped crystals (3). Characterization data for 3 (4 1 knot) 124.2 mg, yield 82%. 1 H NMR (400 MHz, CD 3 OD, ppm, with respect to Cp*Rh): δ = 8.66 (d, J = 5.2 Hz, 8 H, pyridyl-αH), δ = 8.63 (d, J = 2.8 Hz, 8 H, pyridyl-αH), δ = 8.21 (d, J = 8.4 Hz, 4 H, BiBzIm-H), δ = 8.14 (t, J = 8.0 Hz, 4 H, BiBzIm-H), δ = 8.11 (t, J = 7.2 Hz, 4 H, BiBzIm-H), δ = 8.06 (d, J = 8.4 Hz, 4 H, BiBzIm-H), δ = 7.56 (t, J = 12.4 Hz, 4 H, BiBzIm-H), δ = 7.55 (d, J = 2.4 Hz, 4 H, BiBzIm-H), δ = 7.53 (s, 2 H, BiBzIm-H), δ = 7.51 (s, 2 H, BiBzIm-H), δ = 7.39 (m, J = 21.2 Hz, 4 H, BiBzIm-H), δ = 7.27 (d, J = 6.4 Hz, 8 H, pyridyl-βH), δ = 7.13 (d, J = 6.4 Hz, 8 H, pyridyl-βH), δ = 3.52 (dd, J = 14.8, 6 Hz, 8 H, phenyl-H), δ = 2.81 (dd, J = 14.8, 5.2 Hz, 8 H, phenyl-H), δ = 2.12 (dd, J = 17.2, 6 Hz, 8 H, benzyl-H), δ = 1.86 (dd, J = 16.8, 2.8 Hz, 8 H, benzyl-H), δ = 1.76 (s, 60 H, Cp*-H), δ = 1.68 (s, 60 H, Cp*-H). 13 C{ 1 H} (101 MHz, CD 3 OD, ppm): δ = 9.81 (Cp*), δ = 9.96 (Cp*), δ = 98.72(Cp*), δ = 98.79(Cp*), 43.47, 44.28, 117.26, 117.73, 118.46, 120.30, 123.47, 123.93, 124.87, 124.98, 125.08, 125.34, 125.56, 126.24, 128.68, 134.58, 136.26, 142.22, 144.53, 144.80, 145.04, 145.13, 154.50, 154.75, 157.27, 157.43, 164.43, 165.59. IR (KBr disk, cm −1 ): v = 1665, 1620, 1546, 1492, 1420, 1279, 1226, 1161, 1063, 1032, 855, 765, 640, 575, 518, 472. Anal. Calcd for C 224 H 224 F 24 Rh 8 N 32 O 32 S 8 (M = 5047.95): C, 53.30; H, 4.47; N, 1.66. Found: C, 53.32; H, 4.43, N, 1.69. Synthesis of 3′ (Cp*Ir-based figure-eight knot) AgOTf (123.2 mg, 0.48 mmol) was added to a solution of [Cp*IrCl 2 ] 2 (96.0 mg, 0.12 mmol) in CH 3 OH (16 mL) at room temperature. The reaction mixture was stirred in the dark for 24 h and then filtered. BiBzIm (28.0 mg, 0.12 mmol) was added to the filtrate. The mixture was stirred at room temperature for 12 h to give a yellow solution. L2 (41.6 mg, 0.12 mmol) was then added. The mixture was stirred at room temperature for another 12 h to give a yellow solution. The solvent was concentrated to about 8 mL. Upon the addition of diethyl ether, a yellow solid was precipitated and collected. The product was recrystallized from a CH 3 OH/diethyl ether mixture to afford a block-shaped crystal 3′. 145.2 mg, yield 84%. Synthesis of 5 ([2]catenane) AgOTf (123.2 mg, 0.48 mmol) was added to a solution of [Cp*RhCl 2 ] 2 (74.0 mg, 0.12 mmol) in CH 3 OH (20 mL) at room temperature. The reaction mixture was stirred in the dark for 24 h and then filtered. 2,7-Dihydroxybenzo[ lmn ][3,8]phenanthroline-1,3,6,8-(2 H,7 H)-tetraone (DHNDI) (35.6 mg, 0.12 mmol) and NaOCH 3 (12.8 mg, 0.24 mmol) were added to the filtrate. The mixture was stirred at room temperature for 24 h to give a dark red solution. L1 (41.6 mg, 0.12 mmol) was added to the filtrate. The mixture was stirred at room temperature for another 24 h to give a dark red solution. The solvent was concentrated to about 8 mL. Upon addition of diethyl ether, a dark red solid precipitated and was collected. The product was recrystallized from a CH 3 OH/diethyl ether mixture to afford a dark red solid. 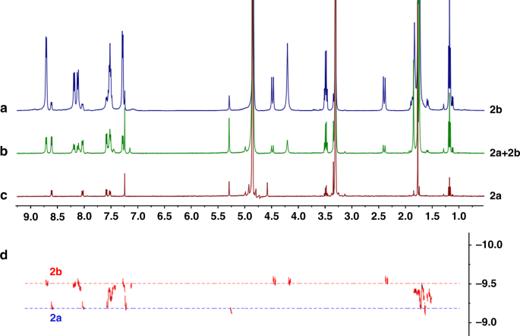Fig. 3 1H NMR spectrum (400 MHz, CD3OD) of2b(a),2a+2b(b), and2a(c). DOSY spectrum (500 MHz, CD3OD) of2a+2b(d), (The peaks at 3.50 and 1.18 ppm belong to diethyl ether) Characterization data for 5 158.4 mg, yield 93%. 1 H NMR (400 MHz, CD 3 OD, ppm): δ = 8.78 (d, J = 4.8 Hz, 8 H, pyridyl-αH), δ = 8.65 (br, 4 H, NDI-H), δ = 8.55 (br, 4 H, NDI-H), δ = 7.92 (d, J = 5.2 Hz, 8 H, pyridyl-βH), δ = 7.30 (s, 8 H, phenyl-H), δ = 5.60 (br, 4 H, benzyl-H), δ = 5.10 (br, 4 H, benzyl-H), δ = 1.81 (s, 60 H, Cp*-H). 13 C{ 1 H} (101 MHz, CD 3 OD, ppm): δ = 7.32 (Cp*), 95.39 (d, J = 9.2 Hz, Cp*), 21.62, 66.75, 123.75, 125.35, 128.91, 130.49, 131.43, 135.89, 140.37, 151.61, 162.91. IR (KBr disk, cm −1 ): v = 1731, 1627, 1585, 1552, 1502, 1458, 1418, 1380, 1266, 1225, 1158, 1123, 1059, 1031, 999, 982, 766, 751, 700, 639, 559, 518, 467. Anal. Calcd for C 112 H 100 F 12 Rh 4 N 8 O 32 S 4 ( M = 2836.14): C, 47.40; H, 3.55; N, 3.95. Found: C, 47.22; H, 3.60, N, 3.78. 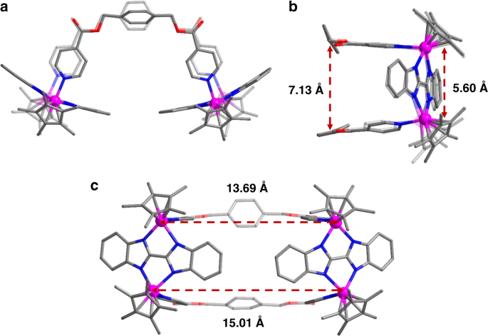Fig. 4 Single-crystal X-ray structure of2a. Top view (a), side view (b), and front view (c). Counteranions and hydrogen atoms are omitted for clarity (N, blue; O, red; C, gray; Rh, purple) 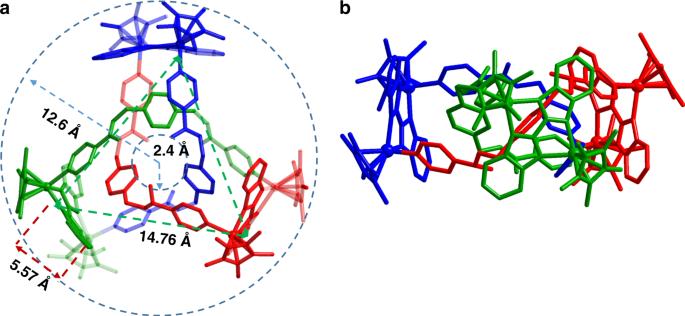Fig. 5 Single-crystal X-ray structure of2b. Top view (a) and side view (b). Counteranions and hydrogen atoms are omitted for clarity 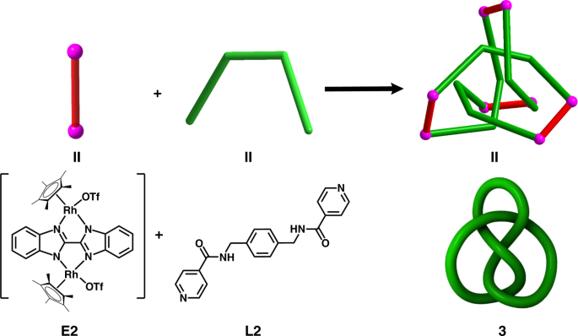Fig. 6 Synthesis of octanuclear figure-eight knot3. Schematic representation of the synthesis of3;The stick model (top) and schematic representation (below) ofE2andL2; The stick model (top) and simplified image of3 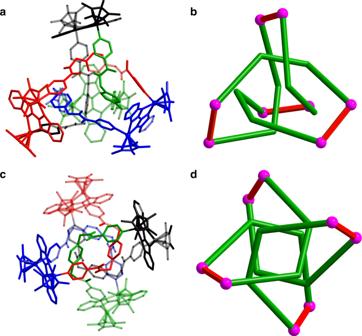Fig. 7 Single-crystal X-ray structure of3. The reduced representation with four crossings (a) and the four-fold symmetry representation (c) of3, and simplified structures of the reduced representation with four crossings (b) and the four-fold symmetry representation (d) of3in which sticks connect the rhodium centers 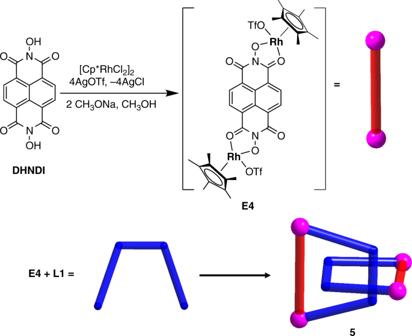Fig. 8 Synthesis of [2]catenane complex5. Schematic representation of the synthesis ofE4(top) and stick model of5(below) 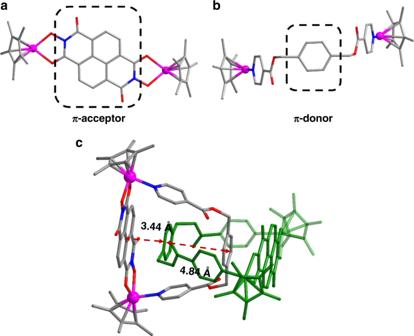Fig. 9 X-ray structure of5([2]catenane).a,bdepictions of the short and long arms (N, blue; O, red; C, gray; Rh, purple) (c) ball-and-stick representations. Counteranions are omitted for clarity ESI-MS: m / z = 2687.20 (calcd for [M–OTf – ] + 2687.18).